Molecular traces of alternative social organization in a termite genome Although eusociality evolved independently within several orders of insects, research into the molecular underpinnings of the transition towards social complexity has been confined primarily to Hymenoptera (for example, ants and bees). Here we sequence the genome and stage-specific transcriptomes of the dampwood termite Zootermopsis nevadensis (Blattodea) and compare them with similar data for eusocial Hymenoptera, to better identify commonalities and differences in achieving this significant transition. We show an expansion of genes related to male fertility, with upregulated gene expression in male reproductive individuals reflecting the profound differences in mating biology relative to the Hymenoptera. For several chemoreceptor families, we show divergent numbers of genes, which may correspond to the more claustral lifestyle of these termites. We also show similarities in the number and expression of genes related to caste determination mechanisms. Finally, patterns of DNA methylation and alternative splicing support a hypothesized epigenetic regulation of caste differentiation. Termites are major pests of human structures, with an annual worldwide cost in damage and control estimated at US$40 B [1] . However, in tropical habitats termites are pivotal for ecosystem function and maintaining biodiversity [2] . Their complex societies have enhanced their environmental adaptability, contributing to their success. Similar to eusocial Hymenoptera (ants, some bees and wasps), termites are characterized by a caste system in which a few individuals reproduce (queens and, in termites, kings) while the large majority (workers and soldiers) perform tasks such as foraging, brood care or defence [3] . Despite these similarities to eusocial Hymenoptera, termite societies have a phylogenetically distinct origin and divergent biological traits. They form a monophyletic clade nested within the Blattodea [4] , indicating a single origin of termite eusociality, whereas eusociality independently evolved multiple times within the Hymenoptera [3] . Termites are hemimetabolous, having several immature stages that become more adult like with each transition, while Hymenoptera have a holometabolous development in which the final larval stage develops via a pupa into adulthood. Despite having distinct lineages with different phylogenetic constraints, termites and eusocial Hymenoptera have evolved similar social and physiological traits. Understanding the selective pressures and specific adaptations necessary to achieve comparable outcomes requires detailed comparisons, particularly at a genetic level. While annotated genomes have been published for seven ant species [5] , [6] , [7] , [8] , [9] , [10] and the honey bee Apis mellifera [11] , sequence data are limited for termites and Blattodea in general. Most termite genetic studies have focused on the development of soldiers with few addressing differences between queens and workers [12] ; therefore, it remains unclear whether eusocial Hymenoptera and termites convergently ‘exploited’ similar mechanisms to achieve similar ends. Here we report the sequence and analysis of the first termite genome of the lower termite Zootermopsis nevadensis nuttingi (Termopsidae), together with genome-wide gene expression data of various caste and developmental stages. We compare these results with previous findings for eusocial Hymenoptera to identify common and divergent associations of traits linked to eusociality. We show significant expansion of gene families related to male reproduction and chemoperception, suggesting differences between Z. nevadensis and eusocial Hymenoptera in mating biology and communication, respectively. We also identify similarities and differences between orders in major gene families that are thought to play a role in the evolution and maintenance of eusociality. These include genes involved in endocrinology, immunity, reproductive development and caste differentiation. Z. nevadensis also exhibits a high level of DNA methylation, which may support a function in regulating phenotypic plasticity, as has been hypothesized for eusocial Hymenoptera. Collectively, the results are an important advance in our ability to elucidate the evolution and mechanistic basis of insect eusociality both within the termites and across taxa. 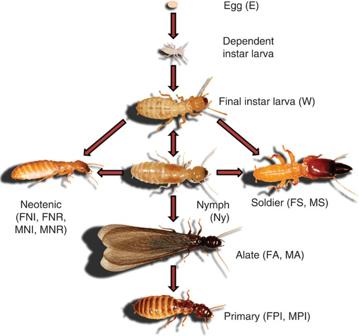Figure 1: Simplified developmental pathway ofZ. nevadensiswith sequenced castes and life stages. Abbreviations indicate (i) sex: female (F) or male (M); (ii) life stage: egg (E), final instar larva without wing buds (hereafter ‘worker’—W), nymph with wing buds (Ny), soldier (S), alate (A), primary (P) or neotenic (N) reproductive; (iii) gonadal activity: currently inactive (I) or reproducing (R). Genome assembly and transcriptomes Genome sequencing utilized a colony consisting of one naturally inbred family with complete homozygosity at four microsatellites that normally have two to three alleles in this population [13] ( Supplementary Note 1 ; Supplementary Table 1 ). After sequencing, reads were strictly filtered leading to an average coverage depth of 98.4 × with an estimated genome size of 562 Mb (Methods; Supplementary Fig. 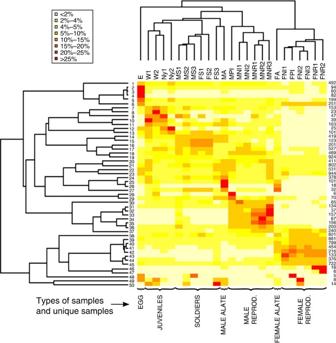Figure 2: Heatmap for the 50-class clustering of RNA-seq transcriptomes. Gene expression, normalized across samples to percentages, ranging from absent (pale yellow) to overexpressed (deep red). Cluster sizes are indicated on the right. Trees at the top and left correspond to hierarchical clusterings of the samples and of cluster-averaged expression, respectively. Type of samples with similar expression patterns (juveniles, soldiers, and male and female reproductives) and unique samples (egg, male and female alates), labelled at the bottom, indicate grouping for differential expression analysis. 1 ; Supplementary Table 2 ). This is the smallest genome known among termites and roaches [14] . 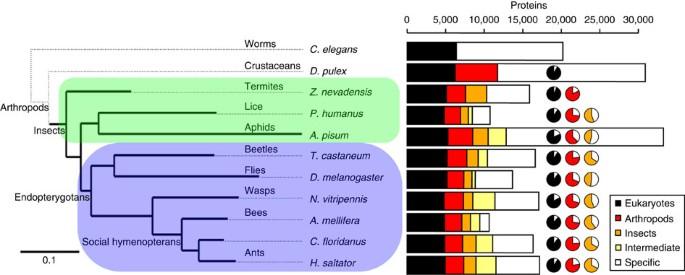Figure 3: Phylogeny and orthology relationships with reference genomes. Tree topology (filled bold line) was obtained by maximum likelihood analysis on proteins. Hemimetabolous and holometabolous species are depicted by a green and blue background, respectively. For each organism, proteins are represented by bars and classified according to orthoMCL analysis: ‘Eukaryote’ clusters withC. elegansand arthropods; ‘Arthropod’ clusters withD. pulexand insects; ‘Insect’ clusters withZ. nevadensisand another insect; ‘Specific’ groups species-specific paralogues and unclustered proteins; ‘Intermediate’ groups all others clustered proteins. Pie charts illustrate each species’ representativeness of the total number of clusters in the categories eukaryote, arthropod and insect. The assembly yielded 93,931 scaffolds, including 85,940 singleton contigs, with an N50 length of 740 kb and a coverage of 493.5 Mb, or 88% of the genome (Methods; Supplementary Table 3 ). Expression analysis of 25 transcriptomes of different sex, developmental stage and caste ( Fig. 1 ; Table 1 ; Supplementary Note 2 ; Supplementary Tables 4 and 5 ) was used to highlight the molecular basis of caste and life stage evolution of Z. nevadensis . We identified gene families that are specifically overexpressed in some castes or life stages ( Fig. 2 ; Methods and Supplementary Note 2.6 ; Supplementary Tables 6 and 7 ). Five of these families were significantly expanded in the termite lineage (see below). Finally, we observed caste-specific expression of orphan genes, that is, genes without any identifiable orthologues, supporting the recently predicted lineage-specific function of orphans [15] . Figure 1: Simplified developmental pathway of Z. nevadensis with sequenced castes and life stages. Abbreviations indicate (i) sex: female (F) or male (M); (ii) life stage: egg (E), final instar larva without wing buds (hereafter ‘worker’—W), nymph with wing buds (Ny), soldier (S), alate (A), primary (P) or neotenic (N) reproductive; (iii) gonadal activity: currently inactive (I) or reproducing (R). Full size image Table 1 Expanded protein families in Z. nevadensis and related families showing significant differential expression. Full size table Figure 2: Heatmap for the 50-class clustering of RNA-seq transcriptomes. Gene expression, normalized across samples to percentages, ranging from absent (pale yellow) to overexpressed (deep red). Cluster sizes are indicated on the right. Trees at the top and left correspond to hierarchical clusterings of the samples and of cluster-averaged expression, respectively. Type of samples with similar expression patterns (juveniles, soldiers, and male and female reproductives) and unique samples (egg, male and female alates), labelled at the bottom, indicate grouping for differential expression analysis. Full size image A total of 15,876 protein-coding genes are reported in OGSv2.2 (Methods; Supplementary Figs 2 and 3 ; Supplementary Table 8 ) with most (95.9%) of them supported by expression data from subsequent transcriptomes. We performed the annotation of the non-coding RNA (ncRNA) and repeated elements (Methods; Supplementary Tables 9–12 ) and predicted protein sequences were functionally annotated using Interpro domains, gene ontology (GO) terms and the Kyoto Encyclopedia of Genes and Genomes (KEGG) database (Methods). Pfam annotation yielded 17,505 predicted domains (3,460 distinct families found in 52% of the termite proteins). Proteins of Z. nevadensis, eight reference insect species, the crustacean Daphnia pulex and a non-arthropod species Caenorhabditis elegans were clustered in orthologue groups, which were used along with functional annotation for genome quality assessment (Methods; Supplementary Note 3 ; Supplementary Tables 13 and 14 ). High orthologue and annotation coverage, despite the deep rooting of the termite lineage in the insect phylogeny (see following section), highlight the quality of the final assembly and gene models ( Fig. 3 ). Figure 3: Phylogeny and orthology relationships with reference genomes. Tree topology (filled bold line) was obtained by maximum likelihood analysis on proteins. Hemimetabolous and holometabolous species are depicted by a green and blue background, respectively. For each organism, proteins are represented by bars and classified according to orthoMCL analysis: ‘Eukaryote’ clusters with C. elegans and arthropods; ‘Arthropod’ clusters with D. pulex and insects; ‘Insect’ clusters with Z. nevadensis and another insect; ‘Specific’ groups species-specific paralogues and unclustered proteins; ‘Intermediate’ groups all others clustered proteins. Pie charts illustrate each species’ representativeness of the total number of clusters in the categories eukaryote, arthropod and insect. Full size image Phylogenetic position of termites Molecular approaches to reconstructing insect phylogeny have been hampered by numerous pitfalls; the rapid radiation of lineages early in the history of insects, compounded with widely varying rates of evolution (as measured by DNA substitutions), and a paucity of comparative genomes from basal insects have resulted in several controversies [16] . Using maximum likelihood and Bayesian approaches applied to sequences of both DNA and translated proteins, we were able to support the basal position of termites, being the outgroup to all other major insect taxa that possess representatives with draft genome sequences ( Fig. 3 ; Methods; Supplementary Figs 4 and 5 ). Previously, only two genomes of hemimetabolous species were available as outgroups to the Endopterygota/holometabola group: Acyrthosiphon pisum (pea aphid) and Pediculus humanus (body louse). These two genomes exhibit features that might bias comparative analysis: substantial fragmentation of the genome sequence, with numerous paralogues and split gene models in A. pisum and a massive genome/proteome reduction owing to a parasitic lifestyle in P. humanus . Unlike these genomes, that of Z. nevadensis has minimal domain fragmentation and a protein number and orthologue/in-paralogue proportion that is in the range for the majority of insect genomes ( Supplementary Note 3 ). These more standard characteristics enhance the value of Z. nevadensis as a third hemimetabolous genome and as a new outgroup to insect genomes. The basal position of the termite genome thus allowed us to test recent hypotheses [17] , [18] regarding the evolution and synteny of the Osiris and Yellow-gene families ( Supplementary Note 4 ; Supplementary Figs 6 and 7 ; Supplementary Table 15 ). These insect-specific families emerged and underwent multiple duplications in the insect ancestor, but orthologues and synteny have then been strongly conserved in all insect genomes. We found that the hemimetabolous Z. nevadensis had orthologues to the Yellow-b and Osiris-1 and -5 subfamilies, which were previously presumed to be specific to Endopterygota/holometabola. We were also able to identify microsyntenic regions that were larger than previously identified in the fragmented and reduced genomes of A. pisum and P. humanus . Comparative genomics reveals gene family expansions Our phylogeny provided the basis for all subsequent genomic analysis to identify species-specific features. Comparative analyses of gene families were conducted to identify major evolutionary changes in the termite genome ( Supplementary Note 5 ; Supplementary Fig. 8 ; Supplementary Tables 16–20 ). When comparing single-copy genes across all sequenced insects, the most notable finding was the absence of several opsin orthologues, the photosensitive proteins used in vision. With only two opsin genes, Z. nevadensis has the smallest repertoire among insects, possibly as a result of principally living in the dark during most of their lifetime. We also found two instances of horizontal gene transfer from entomopathic viruses ( Supplementary Note 5.2 ). Further, we tested gene families for lineage-specific expansion or contraction. Nine families exhibit expansion in Z. nevadensis , the majority being differentially expressed among developmental stages, castes and genders ( Table 1 ). Four related families are not expanded but show similar differential expression across castes ( Table 1 ). These proteins probably play key roles in Z. nevadensis life history, such as mating biology and communication, and are examined in the following sections. Coexpansion of genes related to male fertility Of the gene families that underwent significant expansion in Z. nevadensis , four exhibit a significant male-specific overexpression and have putative associations with male spermatogenesis or cell division ( Table 1 ; Fig. 4 ; Supplementary Note 6 ; Supplementary Figs 9–13 ). Kelch-like protein 10 (KLHL10 with BTB-BACK-Kelch tri-domain) and the seven-in-absentia (SINA) proteins have been associated with E3 ubiquitin ligase complexes involved in protein degradation in spermatids [19] , [20] . Alpha-tubulins interact with SINA during cell division [21] while the human homologue to SINA binds a member of the polycystin ( PKD ) genes that are regularly expressed in testes [22] , [23] . In addition to their expansion, 19 members of the KLHL10 family, and one PKD and one alpha-tubulin show signs of positive selection ( Supplementary Table 16 ). Of note, we found that genes with male-specific overexpression mainly occurred within Z . nevadensis -specific subtrees in each family, with 100% (25 of 25) KLHL10 genes, 67% (4 of 6) SINA genes, 75% (3 of 4) alpha-tubulins and 88% (7 of 8) PKD genes in these specific subtrees being overexpressed in male reproductives. A fifth gene family of extracellular proteases ( ADAMTS , a disintegrin and metalloprotease with thrombospondin motifs), while not significantly expanded in Z. nevadensis , has the largest known copy number among insects suggesting a neofunctionalization in Z. nevadensis . Members of the ADAMTS family and the related ADAM gene family are involved in spermatogenesis [24] , [25] . Four of the five ADAMTS genes are significantly overexpressed in reproductive males. Another significantly expanded gene family, the monodomain Kelch , as well as two non-expanded but significantly differentially expressed families, BTB-Kelch and BACK-Kelch , share domains with KLHL10 genes and may have similar functions. Collectively, the data suggest an expanded role for spermatogenesis regulation in termite evolution. 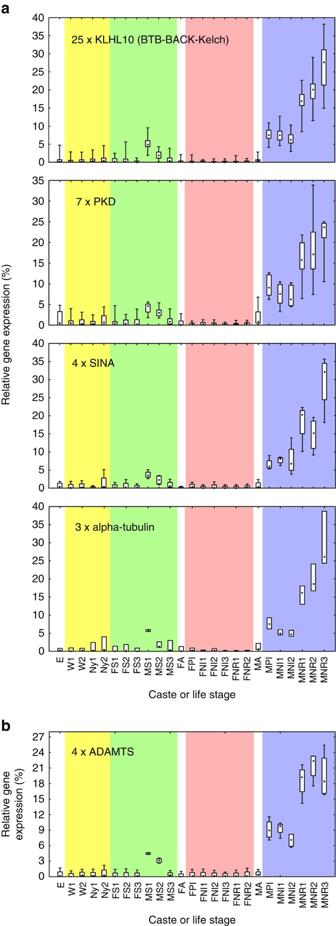Figure 4: Overexpressed genes in male reproductives from select gene families. Relative expression of genes that showed upregulated gene expression in male reproductives and (a) that occurred withinZ. nevadensis-specific subtrees in each gene tree family and that belonged to significantly expanded gene families and (b) that belonged to a gene family with the largest known copy number among insects, but that is not significantly expanded. Expression of individual genes was normalized to 100% across castes and life stages. Medians, 50% intervals and minima/maxima are shown. The number of genes of the respective gene family included for each individual castes or life stages is indicated before the name of the gene family. The procedure to determine the significance of the differential expression of genes and families is detailed in Methods. Genes were significantly overexpressed at false discovery rate <0.05. Yellow bar, workers and nymphs; green bar, soldiers; pink bar, reproductive females; blue bar, reproductive males; for further abbreviations, seeFig. 1. Figure 4: Overexpressed genes in male reproductives from select gene families. Relative expression of genes that showed upregulated gene expression in male reproductives and ( a ) that occurred within Z. nevadensis -specific subtrees in each gene tree family and that belonged to significantly expanded gene families and ( b ) that belonged to a gene family with the largest known copy number among insects, but that is not significantly expanded. Expression of individual genes was normalized to 100% across castes and life stages. Medians, 50% intervals and minima/maxima are shown. The number of genes of the respective gene family included for each individual castes or life stages is indicated before the name of the gene family. The procedure to determine the significance of the differential expression of genes and families is detailed in Methods. Genes were significantly overexpressed at false discovery rate <0.05. Yellow bar, workers and nymphs; green bar, soldiers; pink bar, reproductive females; blue bar, reproductive males; for further abbreviations, see Fig. 1 . Full size image Chemoperception Expansion was also observed in genes pertaining to chemical communication, a crucial component of insect societies [26] . Annotation of the four major gene families involved in insect chemoperception ( Supplementary Note 7 ; Supplementary Figs 14–16 ; Supplementary Tables 21–24 ) identified 336 genes in Z. nevadensis , of which 280 were potentially functional. While this number is much higher than is typically observed in insects, it is intermediate to that of bees and ants [7] , [27] , [28] , reflecting the central role of odorants in eusociality. While the total gene numbers are comparable, their distribution within gene families diverged greatly from what has been observed in Hymenoptera. Odorant receptors (ORs), which confer most of the specificity and sensitivity of insect olfaction, are expanded in ants (344–400) [7] , [9] , [27] and honey bees (163) [28] , but only 69 (63 intact) were found in Z. nevadensis . While the gustatory receptor (GR) repertoire in Z. nevadensis of 87 genes (80 intact) is comparable to that of other social insects (range 10–97 copies), Z. nevadensis shows lineage-specific expansions in different gene subfamilies compared with eusocial Hymenoptera such as the carbon dioxide receptors [7] , [27] , [28] ( Supplementary Note 5.5 ). The ionotropic receptor (IR) family, implicated in gustation and olfaction in Drosophila [29] , is expanded to its greatest known extent in Z. nevadensis , with 150 genes (137 intact). Only 10–32 copies have been observed in eusocial Hymenoptera species [7] , [27] , [28] . The termite IR repertoire includes 13 conserved members present throughout insects, and expansions in three subfamilies of 17, 48 and 66 genes, respectively (corresponding to two domain architectures in Table 1 ). The large difference in the numbers of ORs and IRs provides an opportunity to look at the organization of the olfactory lobe, the first centre for the processing of olfactory information in the insect brain. The antennal lobe is composed of densely packed glomeruli formed from axon terminals projected from receptor neurons in the antennae ( Supplementary Fig. 17 ). Since sensory neurons expressing the same chemoreceptor extend their axons into the same glomerulus, the numbers of olfactory receptors and glomeruli in the insect antennal lobe usually match [30] . Of the 72 olfactory glomeruli of Z. nevadensis estimated based on histological sections ( Supplementary Note 7.5 ), most are probably accounted for by the 63 functional ORs. As a result, only a small number of IRs and GRs can be involved in olfaction, and the remainder must be involved with gustation. The relatively low number of olfactory receptors may indicate that Z. nevadensis has a limited ability to discriminate odours compared with eusocial Hymenoptera. Immunity Parasites and pathogens are generally expected to be important drivers of social insect evolution as their colonial lifestyle creates genetically homogenous populations living in high density, that are ideal targets for infection [31] . Indeed, the decaying wood in which Z. nevadensis lives is also a pathogen-rich environment. To test for a proposed link between eusociality and disease resistance, we analysed immune genes in Z. nevadensis ( Supplementary Note 8 ; Supplementary Fig. 18 ; Supplementary Table 25 ). We identified all of the immune-related pathways described for Drosophila melanogaster and other insects, including pattern recognition, signalling and gene regulation. We found six Gram-negative-binding proteins (GNBPs), which is more than in other insect genomes (maximum of 3 in Nasonia vitripennis ) but fewer than in the crustacean D. pulex (10). Phylogenetic analysis revealed one general insect and five termite-specific GNBPs, supporting the hypothesis that these genes expanded early in isopteran evolution. The termite-specific group includes two GNBPs (GNBP1 and GNBP2) that seem to be under positive selection, at least in some species [32] . Five genes of the immune signalling pathway are significantly overexpressed in female reproductives ( Fig. 5 ) probably indicating that they invest more in immune defence. 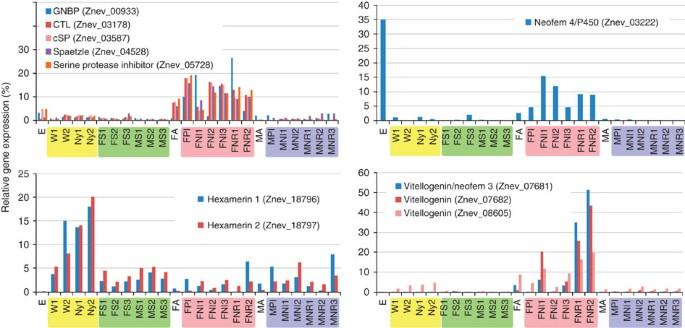Figure 5: Relative expression of several genes implicated in insect immunity, caste differentiation and division of labour. Percent expression is reported for immune-specific genes, hexamerins, P450 and Vgs. All genes are significantly differentially expressed (false discovery rate <0.05, see Methods). Yellow bar, workers and nymphs; green bar, soldiers; pink bar, reproductive females; blue bar, reproductive males. For further abbreviations, seeFig. 1. Figure 5: Relative expression of several genes implicated in insect immunity, caste differentiation and division of labour. Percent expression is reported for immune-specific genes, hexamerins, P450 and Vgs. All genes are significantly differentially expressed (false discovery rate <0.05, see Methods). Yellow bar, workers and nymphs; green bar, soldiers; pink bar, reproductive females; blue bar, reproductive males. For further abbreviations, see Fig. 1 . Full size image We found only three antimicrobial peptides (AMPs): attacin, diptericin and an orthologue of the termite defensin-like gene termicin. This was unexpected, given that an expansion of AMPs in the ant Pogonomyrmex barbatus has been proposed as a response to living in a pathogen-rich environment [7] . However, at least one of the AMPs, termicin, is under strong positive selection in several termite species [32] . These results imply that pathogens play important roles in eusocial insects but that mechanisms to fight these threats differ in a taxon-specific manner. Reproductive division of labour Caste differentiation and a reproductive division of labour is the hallmark of insect eusociality [26] . Proposed regulators of this division in eusocial Hymenoptera include vitellogenins (Vgs), juvenile hormone (JH), biogenic amines and modulators such as JH-binding protein, the insulin/insulin-like growth factor signalling pathway and yellow/major royal jelly protein-like genes. All of these factors appear to interact in complex ways to coordinate development with exogenous cues. We analysed these genes in detail to determine their roles in Z. nevadensis division of labour ( Supplementary Note 9 ; Supplementary Figs 19–28 ; Supplementary Tables 26–32 ) and caste differentiation ( Supplementary Note 10 ; Supplementary Fig. 29 ; Supplementary Table 33 ). Vgs, precursors to the egg yolk protein vitellin, may also be used outside egg production, as they have been seemingly co-opted to help regulate caste determination in honey bees [33] , [34] . We identified four Vgs in Z. nevadensis , two of which seem to be recent duplicates that occur in tandem in the genome and are highly conserved ( Supplementary Note 9.2 ; Supplementary Fig. 19 ). One of these duplications is closely related to Neofem3 , a reproductive-specific gene in three other termite species ( Cryptotermes secundus , C. cynocephalus and Reticulitermes flavipes ) [35] , [36] , [37] , [38] . Three of the four Vg genes, including the recent duplications, were significantly overexpressed in reproducing queens ( Fig. 5 ). One of the Vg genes is also moderately expressed in non-reproductive workers and nymphs ( Fig. 5 ), suggesting it has a function outside oogenesis. This is similar to the expanded functionality observed in duplicated Vgs in the ants Solenopsis invicta and P. barbatus [9] , [39] . In these cases, as with the honey bee, Vg appears to have acquired a role in regulating behavioural caste, and a similar function may have developed in Z. nevadensis . JHs have crucial and diverse functions in insect development, reproduction, longevity and both solitary and social behaviours [40] . Among the known functions of JH in termites are modulation of caste differentiation [12] and adult gonadal activity [41] . JH has different functions at different life stages, and can have multiple functions during the same stage [42] . In Z. nevadensis , we found all crucial enzymes of the JH III biosynthetic pathway and major regulators such as JH-binding proteins ( Supplementary Note 9.3 ; Supplementary Table 27 ). We also found key enzymes in the synthesis of ecdysteroids, another essential hormone group. Unexpectedly, we found neuropeptides normally associated with moulting expressed in reproductives, suggesting a novel function, given that these adults do not moult ( Supplementary Note 9.5 ). Reproductive division of labour is associated with increased longevity of reproductives [43] and various histone-modifying enzymes are implicated in lifespan regulation [44] . In reproductive females, we observed significantly increased expression in two histone deacetylases, sirtuin 6 and 7, and one histone demethylase and other histone-modifying enzymes (see Table 1 and Supplementary Note 9.7 ; Supplementary Figs 21–25 ). Although the lifespan effects of sirtuin 7 are unclear [45] , increased expression of sirtuin 6 leads to prolonged lifespan in male mice [46] . Along with the expression pattern in termites, sirtuins 1 and 6 are more highly expressed in longer-lived reproductive females in the ant Harpegnathos saltator [5] . In honey bees, queen longevity has also been linked to Vg, a possible antioxidant [47] , and the overexpression of this protein in female termite reproductives may play a similar role. In several eusocial insects reproductive division of labour is regulated through cuticular hydrocarbons [48] . In Z. nevadensis , reproductive status is conveyed by an abundance of four long-chained polyunsaturated alkenes [49] . Therefore, we anticipated reproductive-specific expression of genes encoding elongases and desaturases, typically required for their synthesis. Of the 16 elongase and 10 desaturase genes present in Z. nevadensis ( Supplementary Note 9.8 , Supplementary Figs 26 and 27 ), one of each was most highly expressed in the reproductive morphs with highly correlated expression patterns across all samples (Pearson’s correlation: N =25, r 2 =0.93, P <0.00001; Supplementary Fig. 28 ). The reproductive-specific coexpression of these genes makes them candidate regulators of hydrocarbon signalling in Z. nevadensis . Although elongase and desaturase genes involved in hydrocarbon pheromone synthesis have been identified in Diptera [50] , this is the first indication of a similar combined function within the respective pathway in a eusocial insect. Substantial progress has recently been made in the study of the molecular underpinnings of termite caste differentiation [12] . Across various species, several genes, including Cytochrome P450s and hexamerins, have been implicated in caste differentiation. P450s are multifunctional haeme-thiolate enzymes found in all eukaryotes and bacteria. In insects, they contribute to oxidizing endogenous substrates (for example, hormones) and xenobiotic compounds (for example, secondary plant compounds). Members of the CYP4 and CYP15 family have been linked to JH biosynthesis and degradation in insects and termites [12] , [51] , making them promising candidates for caste differentiation regulators. P450s have been linked to JH-dependent termite worker-to-soldier differentiation [12] , and in C. secundus a CYP4 gene, Neofem4 , is specifically upregulated in reproductive females [36] . We found 76 P450 genes in Z. nevadensis , with 55 having at least one complete P450 domain ( Supplementary Note 10.1 ; Supplementary Table 33 ). Members of the CYP4 and CYP6 families each represent about one-third of the total. Their gene number was less than in solitary Diptera ( D. melanogaster : 83, Anopheles gambiae : 111) but intermediate compared with eusocial Hymenoptera (for example, A. mellifera : 46; invasive Argentine ant, Linepithema humile : 111). Of the 69 genes with expression support, 10 were significantly overexpressed in workers and several others also exhibited caste-specific expression patterns, supporting a possible role in caste differentiation. Strikingly, a Neofem4 orthologue is highly expressed in active female reproductives and their eggs ( Fig. 5 ). Hexamerins in solitary insects usually act as storage proteins [52] . We found five hexamerin genes with expression support, four of which were adjacent and probably evolved by tandem duplication ( Supplementary Note 10.2 ; Supplementary Fig. 29 ). The hexamerins sorted into three groups: one grouped with other insects, two were Blattodea-wide/specific and two grouped with hexamerins found in R. flavipes . These latter two are involved in modulating soldier differentiation, probably by controlling JH availability [53] . Specifically, it has been proposed that hexamerins reduce JH availability in workers and nymphal stages, thereby inhibiting soldier development [54] . High hexamerin expression during these relatively plastic stages ( Fig. 5 ) supports this hypothesis. The duplicated genes appear to have been co-opted during termite evolution to function in caste regulation, possibly by acting as a link between nutritional and hormonal (JH) signalling [55] . DNA methylation and alternative splicing We used empirical and computational methods to determine the patterns and roles of DNA methylation in Z. nevadensis ( Supplementary Note 11 ; Supplementary Table 34–38 ; Supplementary Fig. 30 and 31 ). We first identified homologues of DNA methyltransferases 1 and 3, indicating the presence of functional DNA methylation machinery. We then examined depletion of normalized CpG content (CpG o/e), an indicator of DNA methylation within animal genomes [56] . Levels of CpG depletion were 1.5–3 times greater than in other insects [57] , [58] . DNA methylation also preferentially targeted exons and introns ( Fig. 6a ) [57] , [58] . However, depletion of CpG dinucleotides was greater in introns than exons ( Fig. 6a,b ). In addition, DNA methylation in Z. nevadensis targeted the entire length of the gene bodies, except for the first exon following the translation start site, which was subject to lower methylation levels ( Fig. 6b ). Finally, we found a strong correlation between alternative splice events and depletion of CpG dinucleotides. Genes with relatively high methylation levels tended to be alternatively spliced more frequently ( Fig. 6c ). 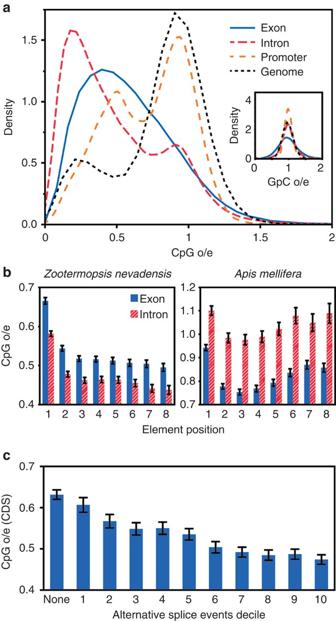Figure 6: Targets and regulatory correlates of DNA methylation inZ. nevadensis. (a) Distributions of CpG o/e for different genomic elements reveals substantial CpG depletion, and thus higher DNA methylation, in introns and exons relative to the genomic background (‘genome’, 1 kb windows) and the region 2 kb upstream of the translation start site (TSS) (‘Promoter’). Inset depicts comparable distributions of GpC o/e, which control for effects unrelated to DNA methylation, such as GC content. (b) Positional CpG o/e of exons and introns inZ. nevadensisandA. melliferarelative to the first eight exons and introns in 5′–3′ orientation from the TSS. (Range innfor element:Z. nevadensis4,349–12,140;A. mellifera2,202–7,756.) (c) InZ. nevadensis, an increasing number of alternative splice events co-occurs with decreasing CpG o/e, suggesting that alternatively spliced genes are preferentially targeted by DNA methylation (P<2.2 × 10−16, the Kruskal–Wallis test,n=2,366 for ‘none’ and 904 for each decile 1–10). Means and 95% confidence intervals are plotted inbandc. Figure 6: Targets and regulatory correlates of DNA methylation in Z. nevadensis . ( a ) Distributions of CpG o/e for different genomic elements reveals substantial CpG depletion, and thus higher DNA methylation, in introns and exons relative to the genomic background (‘genome’, 1 kb windows) and the region 2 kb upstream of the translation start site (TSS) (‘Promoter’). Inset depicts comparable distributions of GpC o/e, which control for effects unrelated to DNA methylation, such as GC content. ( b ) Positional CpG o/e of exons and introns in Z. nevadensis and A. mellifera relative to the first eight exons and introns in 5′–3′ orientation from the TSS. (Range in n for element: Z. nevadensis 4,349–12,140; A. mellifera 2,202–7,756.) ( c ) In Z. nevadensis , an increasing number of alternative splice events co-occurs with decreasing CpG o/e, suggesting that alternatively spliced genes are preferentially targeted by DNA methylation ( P <2.2 × 10 −16 , the Kruskal–Wallis test, n =2,366 for ‘none’ and 904 for each decile 1–10). Means and 95% confidence intervals are plotted in b and c . Full size image Compared with the sequenced genomes of eusocial Hymenoptera, that of Z. nevadensis has both similarities and some profound differences that probably reflect the very different phylogenies and life histories of these species. Among the most pronounced differences was a large expansions in genes associated with spermatogenesis. While males of the eusocial Hymenoptera produce numerous sperm, they usually finish spermatogenesis before completing metamorphosis [59] . Furthermore, males generally die shortly after transferring their gametes to a receptive female. In contrast, termite males complete gamete maturation after their moult, mate repeatedly during their long lives and need to elevate sperm production throughout their lives to meet the growing requirements of an increasingly fecund queen or multiple queens. Such long-term pair bonding with remating is rare among insects [60] . Owing to changing seasonal needs, Z. nevadensis males cyclically activate and deactivate their testes, which may require additional adaptations. The coexpression of expanded genes of the KLHL10, SINA and alpha tubulin families in male reproductives, with potential roles in spermatogenesis, may reflect these added selective pressures on termite males. Another striking difference is the low number of OR genes in Z. nevadensis compared with the eusocial Hymenoptera, which suggests differences in their ability to discriminate volatile substances and communicate with conspecifics. This difference may have evolved as a result of very different nesting behaviours. While Hymenoptera forage away from their nests, encountering a variety of odorants, including those from non-nestmate conspecifics, many of the basal termites, including Z. nevadensis , live their entire lives within a single log [61] . Most of the ants and the honey bee show sophisticated communication behaviour and nestmate recognition, and have an expanded number of ORs relative to Z. nevadensis . We would not expect that all termites have fewer ORs. The ‘higher’ termites, much like ants, have a more sophisticated division of labour, forage outside their nest and exhibit recruitment behaviour [61] . We predict that these species would show an increase in OR genes compared with Z. nevadensis , assuming the expansion of ORs is indicative of communication ability. One area of similarity between the termite and ant genomes is an expansion of genes involved in the production of cuticular hydrocarbons used for communication. Relative to other insects, there is a greater number of desaturase genes in ants [62] , although alkenes or polyunsaturated alkenes have not been found in all ants investigated [63] . Z. nevadensis nuttingi displays two alkadienes and two alkatrienes in the cuticular profile of reproductive individuals [49] , but the number of desaturases is at the lower end of the number of putatively functional desaturase genes found in ants (10–23). If the desaturase genes are linked to more complex communication, we predict that an expansion of desaturase genes should be found in higher termites as we also predicted for genes associated with olfactory perception. There is also evidence that immunity is an important factor in social evolution and that female reproductives invest specifically in immune defence. Compared with solitary insects there are expansions in number of immunity genes for both Z. nevadensis and ants [62] . However, the expansions occurred in different families, possibly as a result of different selective pressures. While the ant P. barbatus has a large number of AMP genes, AMPs are depleted in Z. nevadensis . AMPs may be counter selected to minimize deleterious effects on the microbial symbionts of the termite gut responsible for lignocellulose digestion. In addition, social hygiene and utilization of externalized antibacterial agents can reduce pathogen load in Z. nevadensis [64] , further relaxing selection for more AMPs. We also found evidence supporting the convergent co-option of storage proteins for regulating caste polyphenisms. Just as honey bees appear to utilize Vg to pace caste development via interactions with the endocrine system, termites may use hexamerins, P450s, and possibly Vg, as these families have gone through termite-specific gene duplication and are differentially expressed among castes. Evidence from other termites strongly indicates that hexamerins interact with JH and that a high expression of hexamerins, through interaction with JH, inhibits soldier development [53] , [54] . Vg may play a similar role, although this remains to be tested. A final area of possible similarity between the eusocial insects is in their use of DNA methylation. In Z. nevadensis , the rate of methylation was found to be particularly high relative to other insects [57] , [58] . DNA methylation is involved with gene regulation [65] and alternative splicing [66] , and may be crucial to phenotypic plasticity such as caste differentiation. There is evidence that methylation plays a role in honey bee caste determination, specifically affecting the proportion of brood likely to develop into queens [67] . As has been observed in other insects [57] , [58] , we found methylation primarily in the genic, rather than the intergenic regions of this termite’s DNA. However, unlike the honey bee, methylation was greater in introns than exons ( Fig. 6a,b ). The relative similarity between levels of DNA methylation in introns and exons, as well as the lack of preferential 5′-targeting of DNA methylation ( Fig. 6b ) suggests that patterns of DNA methylation in Z. nevadensis may be more similar to those of basal invertebrate chordates [68] , which exhibit relatively high levels of intragenic DNA methylation compared with those of holometabolous insects [68] . Regardless, the association between alternative splicing and DNA methylation we observed in this termite ( Fig. 6c ) supports the hypothesis that intragenic DNA methylation interacts with messenger RNA splicing to produce an array of phenotypes in eusocial insects [67] , [69] . Collectively, the results of our genome analyses substantially improve our understanding of the mechanisms that have allowed termites to develop and maintain a high degree of social complexity, providing a much needed comparative counterpoint to the wealth of genomic information available for eusocial Hymenoptera. These initial results highlight some of the commonalities and differences that arise from similar needs balanced with phylogenetic and environmental constraints. In addition, having this information for such a basal species greatly facilitates future endeavours to understand the evolution of insects in general. Source of samples Colonies of Z. nevadensis nuttingi were collected in their entirety within wood logs from Pebble Beach near Monterey, California, in November 2010. Species identity of each colony was confirmed by cuticular hydrocarbon analysis using gas chromatography–mass spectrometry. Colonies were transferred to artificial nests consisting of layered precavitated sheets of presoaked spruce ( Pinus glabra ). Nests were kept moist by periodic spraying with distilled water and were maintained in transparent plastic boxes under a 12L:12D light cycle at 20.5 °C. Colony 133 was used to provide all samples for genome sequencing (for additional details see Supplementary Note 1 ). Genome sequencing Sequencing reads were obtained by whole genome shotgun strategy using an Illumina Hiseq 2,000 at the BGI-Shenzhen. Seven paired-end libraries were constructed with insert sizes of 200, 500 and 800 bp, and 2, 5, 10 and 20 kb. DNA samples for genome sequences were derived from soldier heads to minimize contamination with gut content. Fifty heads were extracted for the construction of libraries up to 2 kb, while the DNA from another 150 heads was used for 5–20 kb libraries. In total, we obtained 68 Gb of raw reads. Before assembling, several filtering steps were applied to remove the following: 1 reads with more than 10% of ‘N’ bases or polyA; 2 low-quality reads, with more than 30 low-quality bases (Phred score ≤7); 3 reads with adapter contamination (>10 bp adapter sequence, allowing a maximum of three mismatches); 4 paired reads overlapping each other (>10 bp, allowing 10% mismatch); and 5 PCR duplicates with identical reads between two paired-end reads. The estimated genome size using the 17-nucleotide depth distribution was 562 Mb, which is similar to a previously published estimation. The averaged coverage depth is 98.4-fold and 92% of the bases have more than 20-fold coverage ( Supplementary Fig. 1 ). Statistics are provided in Supplementary Table 2 . Genome annotation The clean reads were assembled by SOAPdenovo into 7,049,535 preliminary contigs covering 396.3 Mbp, of which 613,353 were longer than 100 bp, covering 395.6 Mbp. After scaffolding, these contigs were assembled into 93,931 scaffolds (including 85,940 singleton contigs), yielding a 493-Mb assembly with 21.3 Mb of Ns. The result suggests that the assembly covers 88% of the Z. nevadensis genome, given the estimated genome size of 562 Mb. The scaffold N50 length of the assembly is 740 kb and the contig (continuous fragments extracted from the final assembly) N50 length is 20 kb. More details about contig/scaffold number and length are provided in Supplementary Table 3 . Genome sequence and annotation data are available at http://www.termitegenome.org/?q=consortium_datasets . A genome browser is available at http://www.termitegenome.org/?q=browser . Protein-coding prediction As a first step, three different methods were used to predict gene models: homology-based, RNA-seq-based and de novo . For homology-based gene models, protein sequences from A. mellifera , D. melanogaster , Homo sapiens and two ants ( Camponotus floridanus and H. saltator ) were used. For each of these five species, the prediction pipeline included the following steps: 1 use of TBLASTN ( E -value<1e−5) for homology search; 2 selection of the most similar gene loci when there were multiple candidates; 3 exclusion of regions with identity <50%; 4 use of GeneWise v2.0 to generate gene model structures; and 5 for incomplete gene models, search of 30 bp in the upstream/downstream region to find start/stop codons (7,764 open reading frames (ORFs) completed). Finally, the five homology-based gene predictions were merged into a union set of 20,005 genes (selecting the longest gene models when models overlapped). For RNA-seq data, we built transcriptomes from samples of different life stages or castes of Z. nevadensis (see Supplementary Note 2 ). TopHat v1.3.3 was used to align raw reads against the genome to identify exon–exon splice junctions, and then Cufflinks v0.8.2 was used to reconstruct 1,232,735 transcripts from the spliced alignments. Applying the same merging pipeline as for homology-based predictions to the obtained transcripts resulted in 38,123 gene models with intact ORFs. For de novo prediction, Augustus and SNAP programs were used. After masking the repeats in the genome, 500 genes from homologue-based prediction (with intact ORFs) were selected to train Augustus and SNAP. As a result, 21,224 gene models were predicted by Augustus and 43,140 by SNAP. As a second step, gene models resulting from the three methods were merged into an integrated gene set through multiple filtering steps as follows: 1 RNA-seq gene models were separated into two sets: multiple-exon and single-exon (resp. 11,900 and 26,223 gene models, respectively). As many single-exon genes tend to be incomplete transcripts, we kept the multiple-exon set as the basis of the integrated gene set and subsequent steps were performed to improve the basic set. 2 If more than one gene model of the multiple-exon set overlapped a unique gene model from homology-based prediction, the homology-based model took precedence over the RNA-seq model. 3 Gene models from homology-based prediction not supported by the RNA-seq multiple-exon set but with good homology evidence (Genewise scores ⩾ 80 and CDS length ⩾ 150 bp) were added to the integrated gene set. 4 Single-exon genes from RNA-seq data supported by homology-based prediction, where the homology-based prediction was also a single-exon model, were added to the integrated gene set. 5 Genes from de novo prediction, which did not overlap with any gene in the integrated gene set, were added to the gene set, if they obtain a significant hit (BLASTP E -value<1e−5) to a Swissprot protein. 6 Genes containing transposon-related Interpro domains were removed. 7 Manual curation for some genes of interest was performed using the Apollo Genome Annotation editor [70] . Manual annotations are available at http://www.termitegenome.org/?q=consortium_datasets . We obtained an integrated gene set (named OGS v2.1) of 17,737 gene models ( Supplementary Table 8 ). Most of them have expression support (73%) while just 2.7% are predicted by de novo approaches only ( Supplementary Fig. 2 ). Subsequently, ~1,186 genes were identified as transposon-related genes through Interpro domain annotation and orthoMCL clustering (see below). These genes were not considered in some of the following analyses (for example, the transcriptomics analysis Supplementary Note 2 ), and they were removed from the next gene set release (OGS v2.2—consisting of 15,876 proteins). Finally, the OGSv2.2 contains additional gene models built through manual curation. ncRNA annotation Four types of ncRNAs were annotated in our analysis: transfer RNA (tRNA), ribosomal RNA (rRNA), microRNA and small nuclear RNA ( Supplementary Table 4 ). tRNA genes were predicted by tRNAscan-SE with eukaryote parameters. rRNA fragments were identified by aligning the rRNA template sequences from invertebrate animals to the Z. nevadensis genome using BLASTN with an E -value cutoff of 1e−5. MicroRNA and small nuclear RNA genes were inferred by the INFERNAL software, using release 9.1 of the Rfam database. Repeat annotation The presence of repeats in the genome was examined using two different approaches: First, known transposable elements (TEs) were identified using RepeatMasker (version 3.2.6) against the Repbase. This step identified 13 Mb of known TEs, comprising 2.6% of the genome ( Supplementary Table 5 ). Second, a de novo repeat library was constructed using RepeatScout with default parameters. The generated consensus sequence for each repeat family was then used as reference in RepeatMasker to identify additional high and medium copy repeats (>10 copies) in the genome assembly. This allowed us to identify an additional 119 Mb of repetitive sequences spanning 24.3% of the genome ( Supplementary Table 6 ), consisting primarily of unknown repeats. For non-interspersed repeat sequences, we ran RepeatMasker with the ‘-noint’ option, which is specified for simple repeats, satellites and low complexity repeats. Tandem repeats were also predicted using Tandem Repeat Finder software, with parameters set to ‘Match=2, Mismatch=7, Delta=7, PM=80, PI=10, Minscore=50 and MaxPeriod=12’. In total, repetitive sequences make up 26% of the assembled genome ( Supplementary Table 7 ). Protein functional annotation The function of proteins was predicted using three methods: protein domains, GO and KEGG pathway. Domains are the evolutionary units of protein-coding genes and their emergence and modular rearrangements are strongly associated with adaptive processes that are not always obvious at the gene level. Initial and principal domain annotation was performed using the Pfam database (release 24.0) and HMMER software (version 3.0). Only domains satisfying the Pfam-recommended thresholds (gathering cutoffs) were retained. Overlaps were resolved heuristically by selecting the domain with a strategy based on the best E -value. Additional domains were assigned using Interproscan (v4.3) including SUPERFAMILY, GENE3D, TIGRFAMs, SMART, PROSITE and PRINTS domain models. Proteins were further annotated by GO terms. We created GO annotations with two levels of confidence. The first level is high confidence. Pfam domains and other domains from the previously mentioned databases are annotated by GO terms (pfam2go, smart2go and so on mappings), as well as the Interpro entries (interpro2go). The annotation of a given domain corresponds to the GO terms shared by all annotated proteins possessing this domain (or significantly over-represented for superfamily2go). Hence, when a domain is identified in a protein, the GO annotation of this domain can be safely transferred to that protein. The second level is low confidence. Blast2GO, which is prone to 35% annotation errors, was applied with default values to transfer GO terms significantly over-represented in the best BLASTP hits of termite’s proteins against the NCBI non-redundant database. Note that based on the BLASTP results against the NCBI, we created the list of orphan genes in Z. nevadensis , if no detectable homology ( E -value<10e−3) was obtained. The KEGG Automatic Annotation Server was used to assign proteins to KEGG orthology (KO) groups, using the recommended eukaryote set plus all other available arthropods as references. The KO system is the basis of the KEGG database, since it links annotated proteins to KEGG’s metabolic pathways (PATHWAY) and functional ontology (BRITE). We produced two KO annotation sets: single-best hit was used for preliminary analysis of gene family expansion/contraction, while BBH (bi-directional best hit) was used for preliminary gain-and-loss analysis. Transcriptome analysis Transcriptomes samples were collected from several colonies. Raw reads were aligned on the genome using TopHat. We used edgeR to normalize libraries across samples (trimmed mean of M -values) and to identify differentially expressed genes. Significant over- or underexpression in unique samples without replicates (egg, male alate, female alate) was determined through pairwise comparisons to other types of samples with replicates (juveniles, soldiers, male reproductives, female reproductives), using the DEseq software, with a stringent threshold of 0.01 for the false discovery rate (that is, corrected P values with the Benjamini–Hochberg formula). Differentially expressed genes in types of samples including replicates were identified using the edgeR package with a false discovery rate threshold of 0.05 against all other types of samples and further exclusion of differentially expressed genes in unique samples. From these lists of individual genes, we identified gene families for which a significant number of members, as determined by Fisher’s exact test, were differentially expressed. Expression values for each gene were calculated using the reads per kilo base per million formula. Genes with low expression levels (reads per kilo base per million <5 in all samples) were removed to reduce possible bias. Clustering, using K-means with Euclidean distance was determined with Cluster3.0 and visualized with R. Comparative analysis Domain architectures was used to define protein families and compare the Z. nevadensis protein repertoire with those of D. melanogaster , T. castaneum , N. vitripennis , A. mellifera , C. floridanus , H. saltator , A. pisum , P. humanus and the crustacean D. pulex . Families exhibiting expansion were detected using Fisher’s exact tests (pairwise comparisons of Z. nevadensis with other genomes) on protein domain architecture counts using Pfam, or Interpro for uncovered families ( Supplementary Note 5.5 ). In addition, the OrthoMCL procedure was run using standard parameters on these species and C. elegans to allow a finer perspective over subfamilies ( Supplementary Note 3.2 ). Phylogenetic analysis We conducted phylogenetic analysis to ascertain the position of termites in the evolution of arthropods. Several data sets of orthologous proteins were tested (see below), but the procedure used for phylogenetic reconstructions was the same for each data set: 1 protein sequences were aligned with MAFFT; 2 alignments were cleaned with Gblocks; 3 protein alignments were concatenated into a unique protein superalignment; 4 the underlying DNA superalignment was deduced using only the first two nucleotides of each codon (custom scripts); and 5 four topologies were computed using the two superalignments (nucleotides and amino acids) from two perspectives: a maximum likelihood approach (morePhyML script based on PhyML) and a Bayesian approach (Phylobayes software). For the evolutionary models, we use standard settings, that is the LG+Γ4+I model for morePhyML with amino acids and the GTR+Γ4+I model for nucleotide data, and the GTR+Γ4+CAT model for Phylobayes. Preliminary analyses followed the classical approach for phylogeny at the genome level, that is, we used 2,318 orthoMCL clusters with 1:1 orthologues in the nine arthropod reference species (see Supplementary Table 13 ). However, because of the previously mentioned limitations (the sparse genome sampling and the ancient rapid radiation of lower Neoptera, and the fast evolution of Paraneoptera representatives, especially the pea aphid A. pisum , causing ’long branch attractions’ [LBA]), four different topologies were obtained regarding the relative branching of the termite Z. nevadensis and the Paraneoptera ( P. humanus and A. pisum ). Then, to limit the LBA, several filters were tested including evolution speed (as measured by lowest rates of substitution rates), reduced compositional bias and domain composition. However, none of the filter was successful to obtain an agreement of the four topologies. For secondary analyses, we excluded the D. pulex genome since its position in the tree was already clear while it was likely a burden for the tree reconstruction for several reasons: 1 it is known for its fast evolution (highly adaptive); 2 it contains a large number of paralogues (see also above for D pulex- specific genome features). With likely differential loss of genes, this might produce incorrect 1:1 orthology relationships; 3 we observed that D. pulex has many split gene models (see Supplementary Note 3.4 ), which may probably be misinterpreted as highly derived genes and thus introduce further artefacts; 4 the high phylogenetic distance of this non-insect species from the common ancestor of termites and Paraneoptera might prevent clarification of the ancient rapid radiation of these taxa. We then searched for clear 1:1 orthologues in the expressed sequence tag (EST) data sets of the NCBI non-redundant database. We used reciprocal BLAST best hits with the termite proteins as queries and required a threshold E -value of 10e−50 and a match covering at least 60% of the proteins. We identified three taxa, Diplura, Archaeognatha and Thysanura, offering a common set of 16 orthologous proteins. These taxa are outgroups of Neoptera and belong to the Hexapoda clade ( Supplementary Fig. 4 ). The topologies resulting from this second analysis agreed with the most recently published topologies and the fourth topology had a polytomy that did not contradict the other proposed grouping ( Supplementary Fig. 5 ). How to cite this article: Terrapon, N. et al . Molecular traces of alternative social organization in a termite genome. Nat. Commun. 5:3636 doi: 10.1038/ncomms4636 (2014). Accession Codes: The Whole Genome Shotgun project for the dampwood termite Z. nevadensis has been deposited in the GenBank nucleotide core database under the accession code AUST00000000 . RNA sequencing data have been deposited in the GenBank sequence read archive (SRA) under the accession code SRP022929 .